Potential for interdependent development of tRNA determinants for aminoacylation and ribosome decoding Although the nucleotides in tRNA required for aminoacylation are conserved in evolution, bacterial aminoacyl-transfer RNA synthetases are unable to acylate eukaryotic tRNA. The cross-species barrier may be due to the absence of eukaryote-specific domains from bacterial aminoacyl-transfer RNA synthetases. Here we show that whereas Escherichia coli CysRS cannot acylate human tRNA Cys , the fusion of a eukaryote-specific domain of human CysRS overcomes the cross-species barrier in human tRNA Cys . In addition to enabling recognition of the sequence differences in the tertiary core of tRNA Cys , the fused eukaryotic domain redirects the specificity of E. coli CysRS from the A37 present in bacterial tRNA Cys to the G37 in mammals. Further experiments show that the accuracy of codon recognition on the ribosome was also highly sensitive to the A37G transition in tRNA Cys . These results raise the possibility of the development of tRNA nucleotide determinants for aminoacylation being interdependent with those for ribosome decoding. The accuracy of translating genetic information into protein sequences is important for organismal growth and viability, and depending on the complexity of each organism, it is tightly controlled [1] . In Escherichia coli , the average protein has ∼ 300 amino acids [2] , demanding an error frequency of less than 3×10 −3 per amino acid, which is supported by experimental estimations [3] . In humans, the average protein has ∼ 500 amino acids [4] with many involved in larger complexes, suggesting a need for higher accuracy than that required for E. coli . This demand is likely true for most eukaryotes, where proteins are typically synthesized as longer chains with more complexity. Indeed, the accuracy of protein synthesis in the unicellular eukaryote Saccharomyces cerevisiae is estimated to be ∼ 3-fold higher than that in E. coli [5] . The accuracy of protein synthesis is jointly determined by the aminoacyl-transfer RNA synthetases (aaRS)-catalyzed tRNA aminoacylation and by the ribosome-catalyzed tRNA decoding. Each aaRS synthesizes an aminoacyl-tRNA (aa-tRNA), which enters the ribosome at specific codons for peptide bond formation. In the progressive organismal evolution into higher complexity, how tRNAs, aaRSs, and the ribosome adapted to one another is an important question. Relevant to this question is the frequently observed cross-species barriers to aminoacylation, which block bacterial aaRSs from acylating their eukaryotic tRNAs, despite conservation of the 'identity' nucleotides (for example, the anticodon sequences). The existence of barriers suggests the emergence of eukaryote-specific tRNA determinants possibly to meet the demand for higher accuracy of protein synthesis. Notably, eukaryotic aaRSs are more elaborate than their bacterial counterparts [6] , possessing extension domains in addition to the core domains for aminoacylation. Although the extension domains are not essential for aminoacylation, some can enhance aminoacylation specificity over that of bacterial enzymes [7] . Additionally, eukaryotic ribosomes have expanded from their bacterial counterparts to include new proteins and RNA segments that are implicated in cellular control processes that are unique to eukaryotes. The expansion of both aaRSs and ribosomes in eukaryotes raises the possibility for the development of eukaryote-specific tRNA determinants interdependent on aminoacylation and translation. However, although eukaryotic tRNA nucleotides that act as cross-species barriers have been studied in some cases (for example, tRNA Cys , tRNA Tyr and tRNA Lys ) [8] , [9] , [10] , whether they function to adapt with the expansion of aaRSs and ribosomes has not been tested. Also, while replacement of a bacteria-specific peptide in E. coli TyrRS with a eukaryote-specific peptide from human TyrRS overcomes a cross-species barrier [11] , whether this barrier is linked to the demand for higher accuracy of protein synthesis in eukaryotes is unknown. A cross-species barrier exists in aminoacylation of tRNA Cys . The major determinants for CysRS reside in the U73 nucleotide at the 3′ end of tRNA Cys and in the GCA anticodon [7] , [12] , [13] , both of which are strictly conserved in bacteria, eukarya, and even in archaea [14] , [15] . However, E. coli CysRS (eCysRS) and several other bacterial CysRS, although able to acylate each other's tRNA, are unable to efficiently acylate tRNA Cys in humans [8] , indicating the presence of a eukaryote-specific barrier in human tRNA Cys (htRNA Cys ). The barrier [8] is localized to the tRNA tertiary core and to nucleotide 37 in htRNA Cys . In the tertiary core, whereas htRNA Cys uses the normal Levitt base pair G15–C48 to join the D and variable loops [16] , E. coli tRNA Cys (etRNA Cys ) uses a rare G15–G48 base pair [17] , [18] , which is recognized by eCysRS in an indirect readout mechanism that monitors the backbone structure of the base pair [18] ( Supplementary Fig. S1a,b ). Structural probing shows that the shape of the core in etRNA Cys as defined by the unusual G15–G48 is similar to the shape of the core in other bacterial tRNA Cys using different 15–48 base pairs [19] . At nucleotide 37, the base is conserved as an A in bacteria and in yeast, but is conserved as a G in higher eukaryotes. In the tRNA-bound co-crystal structure [18] , eCysRS only makes contact with the ribose of A37 ( Supplementary Fig. S1c ), indicating another example of indirect readout. However, because the tertiary core and nucleotide 37 are physically separated, whether their indirect readout mechanisms are coupled or independent of each other is unknown. Whereas eCysRS is unable to cross-acylate htRNA Cys , human CysRS (hCysRS) efficiently cross-acylates its bacterial tRNA [8] . The human enzyme shares high homology with eCysRS throughout the core domains [18] , but contains three eukaryote-specific extensions, of which only the C-terminal extension (CTE) is broadly conserved in eukaryotes. The CTE enhances aminoacylation specificity of hCysRS relative to eCysRS [7] , suggesting that it may mediate the transition of the translational apparatus from bacteria to humans. Here we present a comprehensive analysis of the human CTE and its role in the development of eukaryote-specific tRNA determinants interdependent on aminoacylation and ribosome decoding. The analysis consists of the construction of a CTE-fused eCysRS, demonstrating that the fusion overcomes the barrier at both the tertiary core and at nucleotide 37, and the analysis of eukaryote-specific nucleotides for tRNA selectivity on the ribosome, demonstrating that G37 in htRNA Cys imparts increased selectivity relative to A37 in etRNA Cys at both the initial selection and proofreading stages. We also show that G37 has become a eukaryote-specific major determinant of aminoacylation, illustrating a principle of interdependent development of G37 required for both aminoacylation and ribosome decoding. We suggest that this interdependency can increase the accuracy of protein synthesis in eukaryotes relative to bacteria, and that it has implications for the maintenance of the genetic code stability in eukaryotes. Fusion of eCysRS overcomes the cross-species barrier A fusion protein 'eCysRS+CTE' was created, in which the sequence of eCysRS was extended at the C-terminus with the sequence of the human CTE. This fusion markedly improved aminoacylation of htRNA Cys by eCysRS, elevating the catalytic efficiency k cat / K m from ∼ 600-fold below to ∼ 30-fold below that observed with hCysRS ( Fig. 1a,b ; Supplementary Table S1 ). The improvement of activity by the fusion was even more pronounced in single turnover assays, where the effect of the fusion on the aminoacylation rate constant ( k chem ) and on the tRNA affinity constant ( K d ) was significant. Analysis of k chem / K d showed that the fusion increased aminoacylation of htRNA Cys by eCysRS from ∼ 700-fold to ∼ 10-fold below that observed with hCysRS ( Fig. 1c ). In both assays, the fusion protein acted similarly to hCysRS by retaining full activity to aminoacylate etRNA Cys . 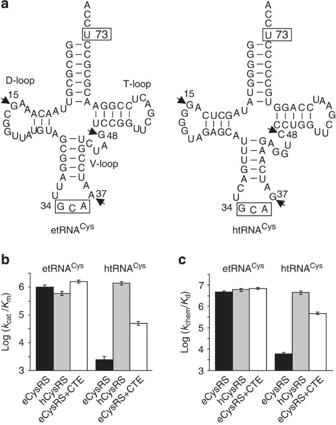Figure 1: Aminoacylation of tRNACyswith cysteine. (a) Sequences of transcripts of etRNACysand htRNACys, showing the conserved U73 and GCA anticodon for aminoacylation and the non-conserved determinants at position 15–48 in the tertiary core and at base 37 in the anticodon loop. (b) Steady-state activity (kcat/Km) of aminoacylation of etRNACysand htRNACysby CysRS enzymes. (c) Single turnover activity (kchem/Kd) of aminoacylation of etRNACysand htRNACysby CysRS enzymes. Data are shown in a logarithmic scale and are the average of 3 determinations. Error bars represent standard deviations. Figure 1: Aminoacylation of tRNA Cys with cysteine. ( a ) Sequences of transcripts of etRNA Cys and htRNA Cys , showing the conserved U73 and GCA anticodon for aminoacylation and the non-conserved determinants at position 15–48 in the tertiary core and at base 37 in the anticodon loop. ( b ) Steady-state activity ( k cat / K m ) of aminoacylation of etRNA Cys and htRNA Cys by CysRS enzymes. ( c ) Single turnover activity ( k chem / K d ) of aminoacylation of etRNA Cys and htRNA Cys by CysRS enzymes. Data are shown in a logarithmic scale and are the average of 3 determinations. Error bars represent standard deviations. Full size image The fusion protein provided a simpler model than the full-length hCysRS to address how the CTE removes the cross-species barrier for eCysRS. Using htRNA Cys as the substrate, we tested if the fusion protein recognized the eukaryote-specific nucleotides in a way that paralleled hCysRS. We showed that the determinants in htRNA Cys that are conserved in etRNA Cys lack such differentiation among the three enzymes. For example, the conserved U73 is the most important nucleotide for tRNA aminoacylation with cysteine [7] , [8] , whose substitutions are typically discriminated by CysRSs by 10 4 –10 5 -fold based on the k cat / K m ratio for wild type (wt) over mutant tRNAs. Indeed, eCysRS, hCysRS, and the fusion protein all strongly discriminated against the U73A mutation, showing discrimination factors of 2.0, 16 and 7.2×10 4 , respectively ( Fig. 2a , Supplementary Table S2 ). The degrees of discrimination by the three enzymes is similar, confirming that U73 is not unique to htRNA Cys . G34 of the conserved anticodon is the second most important nucleotide for aminoacylation [7] , whose mutations are typically discriminated by 10 2 –10 3 -fold. Analysis of the G34C mutation showed similar discrimination by eCysRS and by the fusion protein (2.0 and 2.9×10 3 , respectively), but much greater discrimination by hCysRS (27×10 3 ) ( Fig. 2b ). The weak discrimination by the bacterial and fusion enzymes indicates that they recognize G34 similarly and that G34 is not a eukaryote-specific nucleotide. 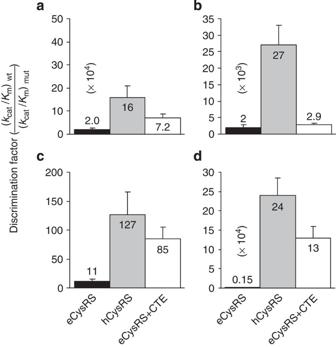Figure 2: Discrimination against mutations in htRNACys. (a) Discrimination against the U73A mutation. (b) Discrimination against the G34C mutation. (c) Discrimination against the G15-G48 mutation. (d) Discrimination against the G37A mutation. Data were obtained by analysis of the steady-statekcat/Km. Each point was the average of 3 determinations, and error bars represented standard deviations. Figure 2: Discrimination against mutations in htRNA Cys . ( a ) Discrimination against the U73A mutation. ( b ) Discrimination against the G34C mutation. ( c ) Discrimination against the G15-G48 mutation. ( d ) Discrimination against the G37A mutation. Data were obtained by analysis of the steady-state k cat / K m . Each point was the average of 3 determinations, and error bars represented standard deviations. Full size image Discrimination of the tertiary core is typically by 10–100-fold [7] , [20] , [21] . Alteration of the normal G15–C48 in the human core to G15–G48 was discriminated by 11-fold by eCysRS, 127-fold by hCysRS, and 85-fold by the fusion protein ( Fig. 2c ). The close similarity between hCysRS and the fusion enzyme indicates that the latter had captured the ability of hCysRS to more strongly recognize the G15–C48 base pair than eCysRS. Similarly, discrimination of the G37A mutation in the anticodon loop of htRNA Cys was 0.15×10 4 -fold for eCysRS but much stronger, 24 and 13×10 4 -fold, for hCysRS and the fusion enzyme ( Fig. 2d ), indicating that the human and fusion enzymes behaved similarly with an ∼ 100-fold higher discrimination relative to eCysRS. Together, these results showed that the fusion enabled eCysRS to recognize the human-specific tertiary core and G37 of htRNA Cys . Additionally, mutational analysis of G37 revealed that the level of discrimination against the G37A mutation by hCysRS and the fusion protein is as strong as that against the U73A mutation (16×10 4 -fold, Fig. 2a,d ), suggesting that G37 has emerged as a eukaryote-specific key determinant equally important as the conserved U73 for aminoacylation of htRNA Cys . Coordination of the core and G37 in the barrier Additional analysis ( Supplementary Table S3 , Supplementary Fig. S2 ) revealed that the recognition of the core and G37 in htRNA Cys is coordinated by the CTE and that the possession of the CTE conferred upon the human and the fusion enzymes two features absent from eCysRS. First, both hCysRS and the fusion enzyme have the flexibility to also recognize A37 in the context of the E. coli core. Whereas both strongly discriminated against G37A in htRNA Cys (mutant htRNA-hM1), both also acylated the A37-containing etRNA Cys (etRNA-wt) with high efficiency, indicating an ability to recognize G37 in the context of the human core and to recognize A37 in the context of the E. coli core. In contrast, the CTE-lacking eCysRS is unable to recognize G37 when associated with the human core. Efficient aminoacylation of htRNA Cys by eCysRS occurred only after introduction of G37A and extensive remodelling of the human core (mutant htRNA-hM2), the latter of which includes G15-G48 and specific substitutions in the D and variable loops [8] . Second, the CTE in the human and fusion enzymes renders the coordinated recognition of G37 with the human core much stronger than the coordinated recognition of A37 with the E. coli core. Although both the human and fusion enzymes discriminated against G37A in the context of the human core by 10 5 –10 6 -fold (htRNA-wt versus htRNA-hM1), they discriminated against A37G in the context of the E. coli core by only 10 3 -fold (etRNA-wt versus etRNA-eM1). The coordinated recognition is also evident in eCysRS, albeit weaker with only a 10 3 -fold discrimination against A37G in the context of the E. coli core (etRNA-wt versus etRNA-eM1). Together, these results show that the cross-species barrier is associated with coordinated changes of the core and nucleotide 37 in the transition from etRNA Cys to htRNA Cys , and that the CTE is required to accompany this transition in the development from eCysRS to hCysRS. Higher codon selectivity of htRNA Cys than etRNA Cys We next examined the codon selectivity of etRNA Cys and htRNA Cys on the ribosome. The accuracy of codon recognition is governed in two stages ( Fig. 3a ): initial selection and proofreading [22] , [23] , [24] , [25] . Initial selection begins with the entry of an aa-tRNA in a ternary complex with EF-Tu and GTP to the ribosome, allowing the sorting of the tRNA by codon–anticodon sampling. Correct pairing leads to rapid GTP hydrolysis [26] , [27] , [28] , whereas near-cognate pairings hinder GTP hydrolysis and non-cognate pairings are rejected from the ribosome [29] . GTP hydrolysis is irreversible and sets the stage for proofreading, where cognate aa-tRNA is accommodated for rapid peptide bond formation, whereas near-cognate ones are rejected. Because selectivity in both stages is largely controlled by kinetics [22] , [23] , [24] , we used kinetic assays with the E. coli ribosome [22] , [23] , [24] . Mammalian ribosomes have not been developed with such assays. 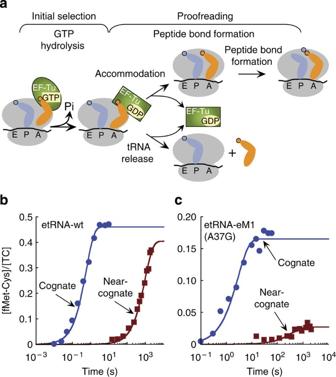Figure 3: Codon recognition on the ribosome. (a) A scheme of codon recognition, showing initial selection of tRNA in the first stage, which is assayed by GTP hydrolysis, followed by proofreading in the second stage, which is assayed by peptide bond formation. (b) Time courses of dipeptide formation on etRNA-wt on UGC (cognate) or CGC (near-cognate) codons measured with a limiting concentration of the ternary complex (0.25 μM). (c) Time courses of dipeptide formation on etRNA-eM1 harbouring the A37G mutation on UGC or CGC codon measured with a limiting concentration of the ternary complex (0.25 μM). Data in (b) and (c) were obtained in single turnover conditions and were well fit to a single exponential equation and plotted on a semi-log scale. Figure 3: Codon recognition on the ribosome. ( a ) A scheme of codon recognition, showing initial selection of tRNA in the first stage, which is assayed by GTP hydrolysis, followed by proofreading in the second stage, which is assayed by peptide bond formation. ( b ) Time courses of dipeptide formation on etRNA-wt on UGC (cognate) or CGC (near-cognate) codons measured with a limiting concentration of the ternary complex (0.25 μM). ( c ) Time courses of dipeptide formation on etRNA-eM1 harbouring the A37G mutation on UGC or CGC codon measured with a limiting concentration of the ternary complex (0.25 μM). Data in ( b ) and ( c ) were obtained in single turnover conditions and were well fit to a single exponential equation and plotted on a semi-log scale. Full size image Selectivity at the initial stage was assayed by the release of Pi from hydrolysis of GTP upon recognition of a cognate codon–anticodon pairing. Each tRNA was prepared by in vitro transcription and used in the form of Cys-tRNA Cys in complex with Tu and GTP. A 70S ribosome with fMet-tRNA fMet in the P site was programmed with a synthetic messenger RNA to place at the A site the cognate codon for cysteine (UGC) or one of three near-cognate (CGC, UAC, UGG) codons. Each complex was rapidly mixed with a purified ternary complex to allow measurement of GTP hydrolysis at 3 μM ribosome ( Table 1 ), which was ∼ 2-fold of the K m of etRNA Cys or htRNA Cys for the ribosome ( Table 2 ). Discrimination of etRNA at the cognate codon ( k app of 13±1 s −1 ) against the second-position and third-position near-cognate codons ( k app s of 0.013±0.003 and 0.033±0.006 s −1 , respectively) was apparent at a level similar to the discrimination reported for other tRNA [30] . However, discrimination against the first-position near-cognate codon (4.5±0.4 s −1 ) was relatively weak. A similar pattern was observed with htRNA, in which the k app for the cognate codon (2.9±0.3 s −1 ) was significantly faster than the k app s for the second-position and third-position near-cognate codons (0.0022±0.0004 and 0.010±0.003 s −1 , respectively), but only slightly faster than the k app for the first-position near-cognate (0.06±0.01 s −1 ) codons. Notably, whereas both tRNAs were weak at discriminating against the first-postiion near-cognate codon, htRNA was 17-fold more discriminative. Table 1 Discrimination against codon–anticodon mismatches. Full size table Table 2 Kinetic parameters of GTP hydrolysis. Full size table The selectivity of cognate against the first-position near-cognate codon was determined by analysis of k app at increasing ribosome concentrations ( Table 2 ; Supplementary Fig. S3 ). This revealed that the K m of each tRNA on the ribosome was similar, whereas the saturating rate constant k GTP varied. Analysis of the specificity constant k GTP / K m between cognate and near-cognate codons showed that the selectivity of htRNA Cys (ratio of 44) was 7.7-fold higher than the selectivity of etRNA Cys (ratio of 5.7). The lower selectivity of etRNA Cys was not due to the lack of nucleotide modifications in the transcript, because native etRNA Cys increased the selectivity from a ratio of 5.7 to 9.0, still 5-fold lower than the selectivity of htRNA Cys . The modest gain in selectivity with native etRNA Cys may be attributable to the natural modification 2-methylthio-N6-isopentenyl (ms 2 i 6 ) of the A37 base [31] . Higher selectivity of htRNA Cys conferred by G37 To determine whether it was the human core or the G37 being responsible for the higher selectivity of htRNA Cys , two mutants of etRNA Cys were created ( Table 2 ; Supplementary Figs S2 , S4 ): eM1 harboured the single A37G substitution and eM5 harboured additional substitutions to recapitulate features of the human core. The A37G substitution alone elevated the selectivity of etRNA Cys to 57, similar to that of htRNA Cys , whereas the additional substitutions in the eM5 mutant made no further improvement (selectivity of 50). Thus, G37 alone is sufficient to elevate the selectivity of etRNA Cys to that of htRNA Cys . The selectivity exhibited by the A37G substitution in etRNA Cys is 10-fold higher than that of etRNA Cys -wt, an effect similar to others induced by a single nucleotide substitution of tRNA ( Supplementary Table S4 ). We tested the role of G37 in the proofreading stage of decoding by monitoring peptide bond formation. The etRNA Cys -eM1 mutant was chosen for comparison with etRNA Cys -wt, because the mutant had the same sequence context as the etRNA Cys -wt except for the A37G substitution, while showing the same selectivity as htRNA Cys -wt in the GTPase assay. A 70S ribosome with fMet-tRNA fMet in the P site was programmed with a synthetic mRNA to place at the A site the cognate (UGC) or near-cognate (CGC) codon. Each complex was rapidly mixed with a ternary complex to allow measurement of fMet-Cys formation ( Fig. 3b,c ; Table 3 ). At the cognate codon, the apparent rate constant ( k app ) of etRNA-wt (1.6±0.2 s −1 ) was similar to the values measured by others [24] , [32] , while the k app of the eM1 mutant (0.31±0.06 s −1 ) was slower. At the near-cognate codon, the k app of etRNA-wt (0.0011±0.0001 s −1 ) was substantially decreased and the value of the mutant was too low to be precisely determined. Table 3 Kinetics of peptide bond formation. Full size table Selectivity of proofreading was determined from the amplitude of dipeptide formation per ternary complex loaded to the ribosome [23] , [24] , [33] , [34] . The selectivity of etRNA-wt at the cognate codon (0.46) and near-cognate codon (0.40) was similar, indicating that discrimination did not occur at the peptide formation step for the wt tRNA. In contrast, the selectivity of the etRNA-eM1 mutant at the cognate codon (0.17) was more than 5-fold greater than at the near-cognate codon (0.03). Thus, the mutant exhibited discrimination at a step where the wt tRNA was incapable of discrimination. From the ratio between the cognate and near-cognate values, the selectivity of proofreading was 1.2 for etRNA-wt and 5.7 for etRNA-eM1, demonstrating a 4.8-fold increase in fidelity of the mutant. The overall selectivity improvement of the eM1 mutant relative to etRNA-wt, calculated as the product of the improvement in the initial selection (10-fold) and in the proofreading ( ∼ 5-fold), was ∼ 50-fold. Using the cross-species barrier of cysteinylation of tRNA as a framework, we have provided a first line of evidence supporting the hypothesis that, due to the expansion of the translational apparatus that accompanies organismal development, the tRNA component of the apparatus has developed discrete determinants interdependent on aminoacylation and decoding. The cross-species barrier in htRNA Cys is localized to the G15-C48 tertiary core and to the mammal-specific G37 in the anticodon loop. Fusion of eCysRS with the human CTE overcomes the barrier at both regions and, more importantly, it redirects the landscape of tRNA recognition such that G37 has become a major determinant for aminoacylation, as important as the conserved U73. The significance of G37 to the fusion protein far exceeds the significance of A37 to the bacterial enzyme. Using the E. coli ribosome, we then showed that the single A37G transition in etRNA Cys confers a 10-fold increase in initial selectivity and an additional 5-fold increase in proofreading, indicating the capacity for a 50-fold increase in the overall accuracy of decoding. The increase in initial selectivity by the A37G mutation is demonstrated in tRNA transcripts. In their native forms, A37 in etRNA Cys is modified to ms 2 t 6 A37, and G37 in htRNA Cys is modified to m 1 G37. Both modifications can further increase tRNA selectivity on the ribosome [35] , suggesting that the higher accuracy displayed by htRNA Cys relative to etRNA Cys in the transcript form should maintain in the native form. We were unable to assess decoding accuracy of the two tRNAs using rabbit reticulocyte ribosome, and we considered yeast ribosome unsuitable, because it presumably co-adapted with yeast tRNA Cys , which harbours A37. However, because the nucleotides that control accuracy of decoding in the ribosome are strictly conserved, the results with the E. coli ribosome strongly suggest that the A37G transition will confer higher selectivity on the human ribosome. Crystal structures of bacterial ribosomes reveal that the accuracy of initial selection is controlled by an induced-fit process of the 30S, involving three strictly conserved nucleotides in the 16S rRNA to closely monitor the geometry of codon–anticodon interactions [26] , [36] , [37] . The three conserved nucleotides are also implicated in the proofreading stage by monitoring the entire anticodon loop structure of tRNA [38] . Nucleotide 37 is localized in a dense network of interactions between the three conserved nucleotides, suggesting that any change in and around the network can result in rearrangement of the contacts and affect the overall accuracy of decoding. The nature of how the A37G transition in etRNA Cys increases accuracy of decoding is unknown, due to the lack of crystal structures of ribosome–tRNA Cys complexes. The A37G transition may increase accuracy by limiting the rearrangement of the contacts to respond only to cognate codon–anticodon interactions. Although the effect of the A37G transition may depend on the sequence context of the anticodon loop, examples of this transition are abundant in tRNA databases: the frequency of G37 in tRNA increases from 12% in bacteria to 29% in humans, whereas that of A37 decreases from 88 to 70% ( Supplementary Table S5 ), indicating a shift of preference from A37 to G37. Recognition of the A37G transition for aminoacylation requires the CTE, which coordinates the transition with changes of the tertiary core. Without the CTE, the coordination still exists but is 10 3 -fold weaker for eCysRS relative to the fusion protein and hCysRS. Structural modelling suggests that the CTE is well suited to perform the coordination, as it emanates from the terminus of the anticodon-binding domain and can reach up to a solvent-accessible channel between the stem-contact fold and the inner corner of the core. Coordinated recognition by the CTE is mediated by indirect readout and is likely secured by the extensive and complementary enzyme–tRNA interface already present in the eCysRS-tRNA structure [18] . The CTE is unique to eukaryotic CysRS, present from yeast to humans, with no sequence homology to any other protein domains. The specificity of the CTE to CysRS is illustrated by the analysis of a CTE-fusion to eMetRS, a close structural homologue of eCysRS. Whereas the native eMetRS is able to acylate the bacterial but not the eukaryotic tRNA Met , illustrating the existence of a cross-species barrier; the CTE fusion to eMetRS does not overcome the barrier but instead impairs the enzyme activity with bacterial tRNA Met ( Supplementary Fig. S5 ). Our work suggests a model consistent with the A37G transition being interdependent on both aminoacylation and ribosome decoding ( Fig. 4 ). This transition would occur only concomitantly with the development of the CTE in human CysRS as an appendage to the core domains in bacterial CysRS. Using an indirect readout mechanism, the CTE would reach around from the anticodon loop all the way to the top of the tertiary core, where it enforces recognition of the human core. To secure the presence of G37 in humans, the CTE would redirect the human CysRS to adopt G37 as a major determinant for aminoacylation. The absence of the CTE from bacterial CysRSs explains their inability to recognize the A37G transition. 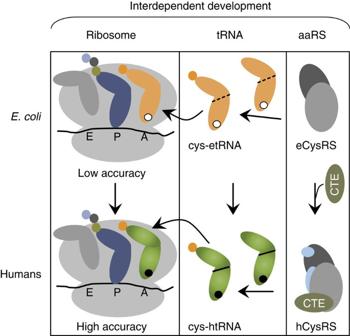Figure 4: A model of interdependent development of tRNACysnucleotides. Centre: The A37G transition (an open circle to a black circle) from etRNACys(orange) to htRNACys(green) is proposed to couple with the transition from the G15-G48 tertiary core (a dashed line) inE. colito the G15-C48 tertiary core (a solid line) in humans. Right: This coupled development is concomitant with the CTE fusion to the core domains of eCysRS (dark grey: activation domain; light grey: tRNA docking domains) to enable recognition of the transition for aminoacylation. The development process also recruits two other eukaryote-specific domains (light blue) to form hCysRS. Left: The A37G transition in the coupled development of tRNA nucleotides confers high codon selectivity on the A site of the ribosome to satisfy the demand for accuracy of protein synthesis in humans. Figure 4: A model of interdependent development of tRNA Cys nucleotides. Centre: The A37G transition (an open circle to a black circle) from etRNA Cys (orange) to htRNA Cys (green) is proposed to couple with the transition from the G15-G48 tertiary core (a dashed line) in E. coli to the G15-C48 tertiary core (a solid line) in humans. Right: This coupled development is concomitant with the CTE fusion to the core domains of eCysRS (dark grey: activation domain; light grey: tRNA docking domains) to enable recognition of the transition for aminoacylation. The development process also recruits two other eukaryote-specific domains (light blue) to form hCysRS. Left: The A37G transition in the coupled development of tRNA nucleotides confers high codon selectivity on the A site of the ribosome to satisfy the demand for accuracy of protein synthesis in humans. Full size image The conservation of A37 in bacterial tRNA Cys has important implications. First, calculation of the error frequency of the A37-bearing etRNA Cys from the k app of dipeptide synthesis at near-cognate (0.001 s −1 ) and cognate (1.6 s −1 ) codons shows a value of 0.6×10 −3 , consistent with the error frequency reported for other bacterial tRNA [24] . At this error frequency, the fidelity of etRNA Cys is sufficient for faithful synthesis of an average protein in bacteria, suggesting that higher accuracy is not necessary. Second, even if the A37G transition had occurred by a single-site nucleotide substitution among bacterial species over time, the resulting tRNA mutant would be unrecognizable to bacterial CysRS, due to the lack of the CTE. Development of the CTE, with more than 100 amino acids in specific structural arrangements, is arguably more difficult than the single nucleotide substitution in tRNA. Third, addition of the CTE to bacterial CysRS is not beneficial, because it would slow down the rate of aminoacylation and incur disadvantage to bacteria. Note that the CTE fusion of eCysRS delays k chem (9.5±0.4 s −1 ) by 2-fold in single turnover assays relative to the unfused enzyme (15.2±0.5 s −1 ), and also delays k cat (0.44±0.02 s −1 ) by 2.5-fold in steady state relative to the control (1.0±0.1 s −1 ). Reduced rates of aminoacylation are harmful to bacteria, particularly during rapid cell growth. In the case of hCysRS, although the native enzyme exhibits a slower k chem (20±1 s −1 ) than a ΔC mutant lacking the CTE ( ∼ 120 s −1 ), there is an advantage in having the CTE, because the specificity of tRNA aminoacylation of the native enzyme is higher than that of the ΔC mutant [7] . Thus, hCysRS would benefit from a trade-off between speed and accuracy by having the CTE. In mitochondria, tRNA Cys is strictly conserved with A37 from yeast to humans and the occurrence of A37 remains stable (25.93% in yeast and 22.22% in humans, Supplementary Table S6 ). In addition, mitochondrial CysRSs consistently lack the CTE, suggesting that aminoacylation of tRNA Cys by these enzymes is operated by a bacteria-like mechanism. Because mitochondrial CysRSs are nuclear-encoded, this bacteria-like mechanism would prevent cross-acylation of the cytosolic G37-bearing tRNA Cys during their transient residence in the cytoplasm before import into mitochondria. The compartment-specific acylation should prevent two enzymes from acylating the same tRNA, a situation that would promote errors and challenge the stability of the genetic code [39] . Cross-species barriers to aminoacylation are widespread among aaRSs. At least for the CysRS enzymes, an interdependent relationship exists between tRNA aminoacylation and tRNA decoding on the ribosome, involving the development of a specific domain in the evolution of CysRS from bacteria to humans. Certainly, analysis of other members of the aaRS family for interdependent relationships of tRNA aminoacylation and decoding will be necessary to gain a broader insight into the evolution of these enzymes and their role in the maintenance of the genetic code stability. Reagents The gene for the eCysRS+CTE fusion protein was generated by inserting the coding sequence of the CTE of hCysRS [7] (from V642 to Q748) into the eCysRS clone [40] at the Bam HI site, such that expression of the fusion extended the C-terminal K461 of eCysRS with the sequence of the CTE. Recombinant His-tagged eCysRS, hCysRS, and eCysRS+CTE were each expressed at 37 °C in BL21(DE3) upon induction with 0.4 mM IPTG and were purified using Talon resin, followed by chromatography through a Mono Q column on an Akta FPLC. Enzyme concentrations were measured by Bradford assay with BSA as the standard, and corrected by active site burst assay [41] . Unmodified transcripts of tRNAs were prepared by in vitro transcription with T7 RNA polymerase from DNA templates generated by primer extension of overlapping olignucleotides. After denaturing gel purification and ethanol precipitation, tRNA transcripts were determined for concentration by absorption at 260 nm and by plateau charging. Tight-coupled ribosomes were prepared from E. coli MRE600 cells, whereas E. coli His-tagged EF-Tu, IF1, IF2, and IF3 were affinity purified [42] . The mRNA sequence for translation was the 022 sequence, encoding 5′-GGG- AAG-GAG -GUA-AAA- AUG -XXX-GUU-CTA-UAC-AAG-ACU-CAC-CAC-CAC-CAC-CAC-3′, where the underline and boldface letters indicate the Shine-Delgarno sequence and the initiation codon, respectively, and XXX indicates the triplet sequence of the cognate and near-cognate codons for cysteine. This sequence was chosen because its initiation region confers high expression levels in E. coli [43] . Each mRNA was synthesized by in vitro transcription from a T7 promoter. Aminoacylation Steady-state assays [40] were performed at 37 °C in a buffer containing 20 mM Tris–HCl, pH 7.5, 20 mM KCl, 10 mM MgCl 2 , 25 mM DTT, 2 mM ATP, 50 μM 35 S-cysteine with 0–120 μM tRNA, and 0–4 nM of CysRS. The K m (tRNA), k cat , and k cat / K m values for each tRNA and enzyme were derived from fitting the data to Michaelis-Menten equation. The k cat / K m data for the G37A mutant was estimated from initial rate of aminoacylation under sub- K m concentrations of the tRNA substrate (40 μM) with 10 μM enzyme. Single-turnover assays were performed similarly but with CysRS in excess of tRNA [44] on the RQF-3 KinTek instrument. GTP hydrolysis GTPase reactions were performed with 7 mM MgCl 2 , which was intermediate between 3.5 mM MgCl 2 of HiFi buffer and 20 mM MgCl 2 of LoFi buffer [23] . This buffer was chosen because it conferred higher stoichiometry in complex formation and faster rates compared with the HiFi buffer. Ternary complex was formed by activating 2 μM EF-Tu with 8 nM γ- 32 P-GTP (6,000 C i /mmole) for 15 min at 37 °C after which Cys-tRNA Cys was added to 1.0 μM and the incubation continued for 15 min at 4 o C. Free GTP was removed from the ternary complex by a Centrispin-20 spin. The 70S Initiation complex (70SIC) was formed by incubating 1–6 μM 70S ribosome with a 1.5-fold molar excess of IF1, IF2 and IF3 and a 2-fold excess of native fMet-tRNA fMet and mRNA with 1 mM GTP for 25 min at 37 °C. Titration of initiation factors relative to the ribosome showed a consistent stoichiometry of 0.7 for fMet-tRNA fMet bound per ribosome. Titration of a ternary complex relative to the 70SIC also showed a stoichiometry of 0.7 for each complex per 70SIC. Aliquots of the mixture of a ternary complex and 70SIC were quenched in acid, followed by reaction with sodium molybdate, and extraction with ethyl acetate [42] . Analysis of k app versus ribosome concentration was fit to a hyperbola (R 2 > 0.98) to yield K m and k GTP . Assays with native etRNA Cys were performed with a crude mixture of E. coli tRNAs isolated from an over-producer strain that generated Cys-etRNA Cys as 5–7% of total tRNA. The strong affinity of EF-Tu for aa-tRNA over tRNA provided the selectivity for loading Cys-etRNA Cys to the ribosome. Native fMet-tRNA fMet was prepared similarly, except that aminoacylation with MetRS was done in the presence of methionyl formyl transferase and N 10 -formyltetrahydrofolate. Peptide bond formation Assays were performed in Buffer A (50 mM Tris-HCl, pH 7.5, 70 mM NH 4 Cl, 30 mM KCl, 7 mM MgCl 2 , and 10 mM DTT). An initiation complex 70SIC (1.0 μM 70S ribosome, 1.5 μM IF1, IF2 and IF3, 1.0 μM 35 S-fMet-tRNA fMet , 2 μM mRNA and 1 mM GTP in Buffer A) was mixed with a ternary complex (1 μM EF-Tu, 0.5 μM Cys-tRNA Cys and 1 mM GTP in Buffer A) at 25 °C. Aliquots were quenched in acid and analysed by electrophoretic TLC [45] . The fraction of 35 S-fMet converted to dipeptide was plotted as a function of time. Single exponential fitting of the plots yielded apparent rate constants for peptide bond formation. If reactions were in multiple turnover conditions, the data would not fit to a single exponential equation. The slow reactions at the near-cognate codon were not due to recycling of Cys-tRNA Cys , because once Cys-tRNA Cys left EF-Tu-GTP, it could not rebind to EF-Tu, which would have hydrolyzed GTP to GDP in the absence of a bound aa-tRNA [46] . Neither were the slow reactions at the near-cognate codon due to hydrolysis of Cys-tRNA Cys , which would have shown the same plateau level for both the wt and eM1 mutant tRNA. How to cite this article: Liu, C. et al . Potential for interdependent development of tRNA determinants for aminoacylation and ribosome decoding. Nat. Commun. 2:329 doi: 10.1038/ncomms1331 (2011).